pT305-CaMKII stabilizes a learning-induced increase in AMPA receptors for ongoing memory consolidation after classical conditioning The role of CaMKII in learning-induced activation and trafficking of AMPA receptors (AMPARs) is well established. However, the link between the phosphorylation state of CaMKII and the agonist-triggered proteasomal degradation of AMPARs during memory consolidation remains unknown. Here we describe a novel CaMKII-dependent mechanism by which a learning-induced increase in AMPAR levels is stabilized for consolidation of associative long-term memory. Six hours after classical conditioning the levels of both autophosphorylated pT305-CaMKII and GluA1 type AMPAR subunits are significantly elevated in the ganglia containing the learning circuits of the snail Lymnaea stagnalis . CaMKIINtide treatment significantly reduces the learning-induced elevation of both pT305-CaMKII and GluA1 levels and impairs associative long-term memory. Inhibition of proteasomal activity offsets the deleterious effects of CaMKIINtide on both GluA1 levels and long-term memory. These findings suggest that increased levels of pT305-CaMKII play a role in AMPAR-dependent memory consolidation by reducing proteasomal degradation of GluA1 receptor subunits. There is a huge and increasing body of experimental evidence for the importance of AMPA-type glutamate receptors in synaptic plasticity and learning, in both vertebrate and invertebrate organisms [1] , [2] , [3] , [4] . The most widely investigated mechanisms of AMPA-dependent plasticity are the CaMKII-mediated phosphorylation of GluA proteins, such as GluA1 (refs 5 , 6 ), and the trafficking of AMPARs from the cytoplasm to the post-synaptic density (PSD) [7] , [8] , [9] . Recent work has suggested that lysosomal or proteasomal degradation of ubiquitinated AMPARs is also a key component of the formation of synaptic plasticity [10] , [11] , [12] , [13] . Recently it also has been shown that in dendritic spines, CaMKII, autophosphorylated at Threonin 286 (pT286-CaMKII), acts as a scaffold to recruit proteasomes to the PSD [14] , suggesting another link between CaMKII and AMPARs, via the proteasome, during formation of synaptic plasticity. Agonist-triggered proteasomal degradation of AMPARs is likely to occur shortly after synaptic plasticity has been initiated by the activation of NMDA receptors, when proteasomes are recruited to synapses [15] . However, previous and more recent work has shown that there is also a prolonged upregulation of AMPAR protein levels in LTP and behavioural learning, which is necessary for long-term synaptic plasticity and associative memory, respectively [16] , [17] . The mechanism that acts against the proteasomal degradation of AMPARs and maintains their level is unknown. It is known however that autophosphorylation of CaMKII at Threonin 305 (T305), which follows its early autophosphorylation at T286 (ref. 18 ), promotes the dissociation of CaMKII from the PSD [19] , [20] , [21] . Increased autophosphorylation of CaMKII at T305 is thus likely to lead to a decrease in proteasomal translocation to the PSD and consequently, a decreased degradation of AMPARs in synapses. We therefore hypothesized that after classical conditioning, autophosphorylation of CaMKII at T305 plays an important role in maintaining increased AMPA receptor levels by reducing proteasomal degradation of the GluA1 receptor protein. We tested this hypothesis in an experimental system that offers both a robust single-trial classical conditioning paradigm [22] , [23] and established evidence regarding the role of CaMKII and NMDA receptors in the acquisition and consolidation of behavioural long-term memory [24] . This system is the ganglionic central nervous system of the mollusc Lymnaea stagnalis . In recent years, the role of a number of major evolutionarily conserved molecular pathways involved in the acquisition, consolidation and reconsolidation of memory already have been elucidated in this system, in the context of associative long-term memory (ALTM) in intact animals [23] , [25] , [26] , [27] , [28] , [29] , [30] . Another major advantage of the use of Lymnaea is that after food–reward classical conditioning both the acquisition and storage of the implicit memory trace take place in the buccal and cerebral ganglia [31] , which therefore can be selectively targeted in biochemical and immunohistochemical assays following behavioural training and pharmacological treatment of intact animals. Using a combination of classical conditioning, behavioural pharmacology, immunohistochemistry and western blot assays, here we identify a novel interlinked role for CaMKII and AMPARs in the consolidation of long-term associative memory in Lymnaea . Our findings suggest a role for T305 autophosphorylated CaMKII (pT305-CaMKII) in maintaining increased levels of GluA1 receptors in the face of proteasomal degradation during memory consolidation after classical conditioning. AMPAR activity at 6 h post training is necessary for ALTM Maintained levels of newly synthesized AMPARs have been suggested to contribute to the stabilization of ALTM in mice [17] . Therefore, in our first experiment we tested the hypothesis that AMPARs play a similar role in the consolidation of ALTM in Lymnaea . Specifically, we investigated whether AMPAR activation at 6 h post training was required for the expression of the classically conditioned response to the conditioned stimulus (CS) at 24 h post training, that is, the behavioural readout of ALTM in the paired group. We compared the conditioned response of an AMPAR inhibitor (CNQX)-injected and a vehicle-injected paired group with each other and against the baseline response in a naive group ( Fig. 1 ). Additionally, we used a group of animals that were classically conditioned but not treated with CNQX or vehicle (Paired) and another group of animals (Unpaired) that were subjected to an explicitly unpaired training protocol ( Fig. 1 ). The former of these two groups was used for a comparison with the vehicle-injected group, while the latter served as a control for the associative training protocol used in the experiments. 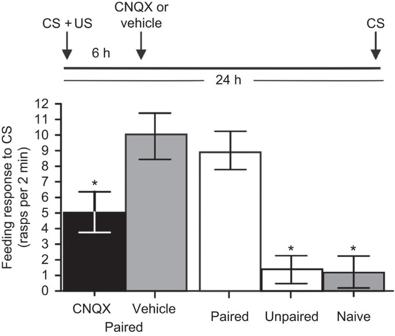Figure 1: GluA1 AMPAR activity is necessary for memory consolidation inLymnaea. Treatment with CNQX 6 h after classical conditioning (CS+US) results in impairment of memory at 24 h after training. Timeline for the experiment is shown above the diagram. When tested with the amyl acetate CS at 24 h, the CNQX-treated classically conditioned animals (N=23) show a significantly lower feeding response compared with the vehicle-treated classically conditioned animals (N=21). Naive animals (N=22) or animals subjected to unpaired training (CS-US interval 1 h,N=20) respond very weakly to the CS. Means±s.e.m. values are shown. Asterisks indicate response levels that are significantly lower than those both in the vehicle-treated and untreated paired (N=19) group, which have virtually identical high response levels. One-way ANOVA,P<0.0002. Tukey’s tests: CNQX (Paired) versus Vehicle (Paired), Naive versus Vehicle (Paired) and Naive versus Paired, allP<0.05; CNQX (Paired) versus Naive, Paired versus Vehicle (Paired) and Unpaired versus Naive, allP>0.05). This experiment was replicated twice. Figure 1: GluA1 AMPAR activity is necessary for memory consolidation in Lymnaea . Treatment with CNQX 6 h after classical conditioning (CS+US) results in impairment of memory at 24 h after training. Timeline for the experiment is shown above the diagram. When tested with the amyl acetate CS at 24 h, the CNQX-treated classically conditioned animals ( N =23) show a significantly lower feeding response compared with the vehicle-treated classically conditioned animals ( N =21). Naive animals ( N =22) or animals subjected to unpaired training (CS-US interval 1 h, N =20) respond very weakly to the CS. Means±s.e.m. values are shown. Asterisks indicate response levels that are significantly lower than those both in the vehicle-treated and untreated paired ( N =19) group, which have virtually identical high response levels. One-way ANOVA, P <0.0002. Tukey’s tests: CNQX (Paired) versus Vehicle (Paired), Naive versus Vehicle (Paired) and Naive versus Paired, all P <0.05; CNQX (Paired) versus Naive, Paired versus Vehicle (Paired) and Unpaired versus Naive, all P >0.05). This experiment was replicated twice. Full size image We found that treatment of classically conditioned animals with CNQX, at 6 h post training resulted in significant memory impairment at 24 h after training ( Fig. 1 ). This finding provided the first experimental evidence for a role AMPARs play in memory consolidation after associative learning in Lymnaea . Vehicle treatment did not impair memory consolidation compared with no treatment and similar to previous findings [22] , [23] , [24] , animals subjected to unpaired training showed no response to the CS ( Fig. 1 ). Increased AMPAR levels at 6 h after reward training Next, we tested the hypothesis that similar to vertebrates [17] , the initial learning-induced activation of NMDA receptors in Lymnaea , which is required for the acquisition of long-term associative memory [24] , is followed by a prolonged increase in the level of AMPARs in circuits involved in the formation and maintenance of behavioural long-term memory. To test this hypothesis we used a combination of behavioural, western blot and immunohistochemical methods. For the latter two methods, we used an antibody against mammalian GluA1 (for the validation of the use of this antibody in Lymnaea see Supplementary Fig. 1 ). First, we used the western blot method to measure total GluA1 levels in the buccal and cerebral ganglia (interconnected by the cerebro-buccal connective) at 6 h after classical conditioning. The samples for these tests were obtained at 6 h post training because a previous study demonstrated a significantly increased number of hippocampal neurons expressing GluA1 AMPA receptor subunits at this time point after fear conditioning in mice [17] . We found that total GluA1 levels were significantly increased at 6 h post conditioning in the samples from the paired as well as the unpaired group of animals compared with the naive controls ( Fig. 2a ), but only the paired group showed a conditioned feeding response at 24 h after classical conditioning ( Fig. 2b ). This initial finding was consistent with the finding in mice that the proportion of GluA1-expressing hippocampal neurons increased after both paired and unpaired training [17] , indicating a close similarity of the underlying molecular mechanisms in invertebrates and vertebrates. 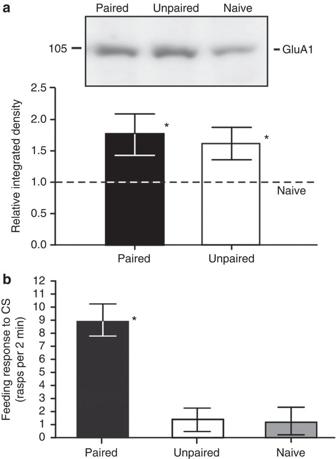Figure 2: Training-induced upregulation of GluA1 AMPA receptors during memory consolidation inLymnaea. (a) A representative example of GluA1 immunoblot bands from a paired, an unpaired and a naive sample, run on the same gel, is shown above the graphs (full-length blot is presented inSupplementary Fig. 7a). Density data obtained from paired (N=8) and unpaired (N=8) samples were normalized to the mean of the density data obtained from naive samples ran on the same gels (N=8), which provided a baseline level of 1 (dashed line). In the graphs means±s.e.m. are shown. Both paired and unpaired training results in significantly increased GluA1 receptor protein levels in the ‘learning’ ganglia at 6 h post training (one-samplet-tests: paired versus naive baseline,P=0.047; unpaired versus naive baseline,P=0.048). There is no statistically significant difference between the GluA1 levels in the samples from the paired and unpaired group (two-tailed unpairedt-test: paired versus unpaired group,P=0.71). Asterisks indicate significant (at leastP<0.05) differences compared with the naive baseline. (b) At 24 h post training, only the paired group (N=19) showed a conditioned response to the CS. Means±s.e.m. of the feeding response to the CS are shown. Naive animals (N=22) or animals subjected to unpaired training (CS-US interval 1 h,N=20) did not respond to the CS (ANOVA,P=0.0001. Tukey’s test: paired versus unpaired,P<0.05, paired versus naive,P<0.05, unpaired versus naive,P>0.05). Asterisk indicates significance compared with both unpaired and naive response levels. These experiments were replicated twice. Figure 2: Training-induced upregulation of GluA1 AMPA receptors during memory consolidation in Lymnaea . ( a ) A representative example of GluA1 immunoblot bands from a paired, an unpaired and a naive sample, run on the same gel, is shown above the graphs (full-length blot is presented in Supplementary Fig. 7a ). Density data obtained from paired ( N =8) and unpaired ( N =8) samples were normalized to the mean of the density data obtained from naive samples ran on the same gels ( N =8), which provided a baseline level of 1 (dashed line). In the graphs means±s.e.m. are shown. Both paired and unpaired training results in significantly increased GluA1 receptor protein levels in the ‘learning’ ganglia at 6 h post training (one-sample t -tests: paired versus naive baseline, P= 0.047; unpaired versus naive baseline, P= 0.048). There is no statistically significant difference between the GluA1 levels in the samples from the paired and unpaired group (two-tailed unpaired t -test: paired versus unpaired group, P= 0.71). Asterisks indicate significant (at least P< 0.05) differences compared with the naive baseline. ( b ) At 24 h post training, only the paired group ( N =19) showed a conditioned response to the CS. Means±s.e.m. of the feeding response to the CS are shown. Naive animals ( N =22) or animals subjected to unpaired training (CS-US interval 1 h, N =20) did not respond to the CS (ANOVA, P= 0.0001. Tukey’s test: paired versus unpaired, P< 0.05, paired versus naive, P< 0.05, unpaired versus naive, P> 0.05). Asterisk indicates significance compared with both unpaired and naive response levels. These experiments were replicated twice. Full size image The mice fear conditioning experiments however also revealed that although the increase in the number of GluA1 containing hippocampal CA1 neurons was similar in the paired and unpaired group, only the paired group showed a learning-associated selective trafficking of newly synthesized GluA1 receptors to mushroom-type dendritic spines of the CA1 neurons [17] . We therefore tested the hypothesis that similar to fear conditioning in mice, a selective increase of the number of newly synthesized GluA1 receptors in post-synaptic structures supports the consolidation of long-term associative memory after reward learning in Lymnaea. To establish the cellular localization of GluA1 immunostaining and its alterations after training, we performed immunohistochemical tests on sections from the buccal and cerebral ganglia of trained (paired and unpaired) and naive animals; in Lymnaea and other molluscs these ganglia contain all the neuronal circuitry involved in food-reward learning [31] , [32] (the ‘learning ganglia’). GluA1 receptors were detected as immunopositive punctae both in the cell bodies of neurons of the feeding system (known to respond to glutamate and AMPA [33] ) and in the neuropile region where most of the synaptic contacts are made between the neurites of neurons (snail neurons do not possess dendrites) ( Fig. 3 ). A quantitative analysis of the confocal images revealed that the majority (between 60 and 64%) of the green and red pixels (representing GluA1 and PSD-95 immunoreactivity, respectively) colocalized and showed a high level of intensity correlation in the buccal and cerebral ganglia as well as separately in both the neuropile and on the periphery of neuronal somata in these two ganglia ( Supplementary Fig. 2 ). 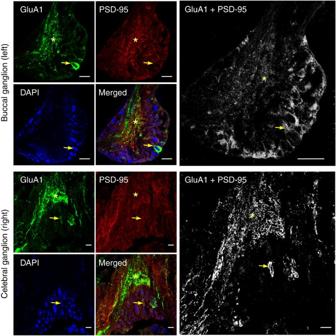Figure 3: GluA1 receptors are present in post-synaptic sites within the ‘learning ganglia’. Colocalization of GluA1 (green fluorescence) and PSD-95 (red fluorescence) in the buccal (top set of panels) and cerebral ganglia (bottom set of panels). The positions of neuronal cell bodies were mapped by using DAPI staining of the nuclei. The neuropile is indicated by an asterisk. The large panels on the right show the distribution of co-localized PSD-95 and GluA1 immunopositive pixels (real size of each pixel, 0.25 μm × 0.25 μm), in both the neuronal cell body region and the neuropile. Arrows indicate examples of neuronal cell bodies with particularly strong colocalization of GluA1 with PSD-95, both in the soma and the axon hillock. Scale bars represent 50 μm. This experiment was replicated three times. Figure 3: GluA1 receptors are present in post-synaptic sites within the ‘learning ganglia’. Colocalization of GluA1 (green fluorescence) and PSD-95 (red fluorescence) in the buccal (top set of panels) and cerebral ganglia (bottom set of panels). The positions of neuronal cell bodies were mapped by using DAPI staining of the nuclei. The neuropile is indicated by an asterisk. The large panels on the right show the distribution of co-localized PSD-95 and GluA1 immunopositive pixels (real size of each pixel, 0.25 μm × 0.25 μm), in both the neuronal cell body region and the neuropile. Arrows indicate examples of neuronal cell bodies with particularly strong colocalization of GluA1 with PSD-95, both in the soma and the axon hillock. Scale bars represent 50 μm. This experiment was replicated three times. Full size image Importantly, after paired, but not unpaired, training, GluA1 expression was significantly increased in both the neuropile and neuronal cell body region, in both the buccal and cerebral ganglia ( Fig. 4 ). These results confirmed that similar to the mouse hippocampus, paired training results in a significant increase in the number of GluA1 receptors in the neurons of the learning circuitry of the Lymnaea CNS. By contrast, the animals subjected to unpaired training did not show an increase in GluA1 levels in the neurons of the ‘learning ganglia’ at 6 h post training ( Fig. 4 ), neither did they show an increased response to the CS at 24 h post training ( Fig. 1 ). Interestingly, in the sections from classically conditioned animals there was also an increased level of GluA1 expression in the buccal commissure ( Fig. 4 ), possibly indicating an increased level of trafficking of GluA1 receptors in the contra-laterally projecting axons of motoneurons and interneurons of the feeding network, from the cell body to presynaptic terminals. 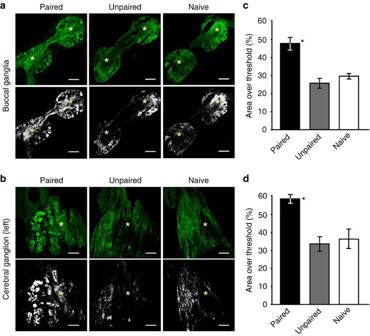Figure 4: Classical conditioning increases the number of GluA1 receptors in the ‘learning ganglia’. (a,b) The top panels in each part show examples of GluA1 immunostaining in sections from the buccal and cerebral ganglia, respectively. The ganglia were dissected at 6 h post training from Paired, Unpaired and Naive animals (N=5 in each group). The bottom panels in each part show the signals in the same sections computed to be above a pre-set 8-bit grey-scale threshold value (65) that was the same for all samples (for details see Methods). Asterisks indicate comparable locations of the neuropile in the samples from paired, unpaired and naive animals. Scale bars represent 100 μm. (c,d) Statistical data obtained by the analysis of all the buccal and cerebral ganglia samples, respectively. The bar diagrams show the % of the area of immunostaining (means±s.e.m.) that exceeds threshold. Asterisk indicates that in both pairs of ganglia this value is significantly greater in the paired group compared against both the unpaired and naive group. (c, One-way ANOVA:P<0.0003. Tukey’s: Paired versus Unpaired and Paired versus Naive,P<0.05; Unpaired versus Naive,P>0.05. (d) One-way ANOVAP<0.001. Tukey’s: Paired versus Unpaired and Paired versus Naive,P<0.05; Unpaired versus Naive,P>0.05). Very similar statistical results were obtained when we analysed the differential expression of GluA1 in the paired and unpaired snail ganglia relative to naive levels (see Methods). This experiment was replicated twice. Figure 4: Classical conditioning increases the number of GluA1 receptors in the ‘learning ganglia’. ( a , b ) The top panels in each part show examples of GluA1 immunostaining in sections from the buccal and cerebral ganglia, respectively. The ganglia were dissected at 6 h post training from Paired, Unpaired and Naive animals ( N =5 in each group). The bottom panels in each part show the signals in the same sections computed to be above a pre-set 8-bit grey-scale threshold value (65) that was the same for all samples (for details see Methods). Asterisks indicate comparable locations of the neuropile in the samples from paired, unpaired and naive animals. Scale bars represent 100 μm. ( c , d ) Statistical data obtained by the analysis of all the buccal and cerebral ganglia samples, respectively. The bar diagrams show the % of the area of immunostaining (means±s.e.m.) that exceeds threshold. Asterisk indicates that in both pairs of ganglia this value is significantly greater in the paired group compared against both the unpaired and naive group. ( c , One-way ANOVA: P <0.0003. Tukey’s: Paired versus Unpaired and Paired versus Naive, P <0.05; Unpaired versus Naive, P >0.05. ( d ) One-way ANOVA P <0.001. Tukey’s: Paired versus Unpaired and Paired versus Naive, P <0.05; Unpaired versus Naive, P >0.05). Very similar statistical results were obtained when we analysed the differential expression of GluA1 in the paired and unpaired snail ganglia relative to naive levels (see Methods). This experiment was replicated twice. Full size image We also compared the GluA1 content of the cerebro-buccal connectives in the same Paired, Unpaired and Naive preparations where GluA1 expression was measured in the neuropile and cell body region of the buccal and cerebral ganglia. This analysis both confirmed that GluA1 receptors are expressed in the cerebro-buccal connectives and showed that their levels are higher in both the Paired and Unpaired group compared with the Naive group ( Supplementary Fig. 3 ). This finding indicates that a possible source of increased GluA1 levels found in the Unpaired samples using the western blotting method was the cerebro-buccal connectives. Another possible source is the connective tissue surrounding the buccal and cerebral ganglia that also shows GluA1 expression in whole-mount preparations ( Supplementary Fig. 3 ), but a quantitative assessment of training-induced changes in this tissue was not possible. CaMKIINtide impairs ALTM and reduces pT305-CaMKII levels Previous experiments have demonstrated that in Lymnaea the consolidation of ALTM requires the synthesis of new proteins for only up to 1 h after single-trial classical conditioning [34] . This implies that the increased levels of GluA1 proteins we detected at 6 h post training must have been synthesized at least 5 h earlier, and somehow maintained since then. Other experiments in vertebrates have demonstrated that AMPARs are subject to ubiquitination-mediated proteasomal degradation [10] , [13] , and more recently, that the recruitment of proteasomes to the PSD is promoted by pT286-CaMKII (ref. 14 ). On the other hand, autophosphorylation of CaMKII at T305 promotes the dissociation of CaMKII from the PSD [19] , [20] , [21] and therefore would be expected to help maintain higher AMPA receptor protein levels by reducing proteasomal recruitment to the GluA1-expressing post-synaptic sites. We therefore investigated whether the same single-trial classical conditioning procedure that resulted in increased AMPA receptor levels at 6 h post training would also lead to an increased level of pT305-CaMKII and whether this increase could be blocked by CaMKIINtide. First, using immunohistochemistry, we found a very high level of colocalization of GluA1 and CaMKII immunostaining in both the buccal and cerebral ganglia ( Fig. 5 ). In alternating sections, we found a close correspondence between the localization of pT305-CaMKII and AMPARs ( Fig. 5 ). However, unlike GluA1 and PSD-95, or GluA1 and CaMKII, the colocalization of GluA1 and pT305-CaMKII could not be investigated in the same sections because we had to use the same secondary antibody for the detection of these two different proteins (see Methods). Furthermore, we found that the immunohistochemical method was not well suited for a quantitative analysis of the combined effects of training and CaMKIINtide on CaMKII phosphorylation levels, because these need to be normalized to CaMKII, whose expression was ubiquitous ( Fig. 5 ), but quite variable. Therefore, we used the western blot method for our quantitative analysis of pT305-CaMKII levels in the ‘learning ganglia’, which allowed us to make more robust statistical comparisons. 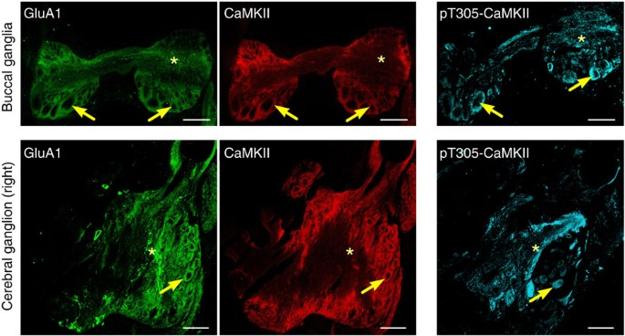Figure 5: Colocalization of GluA1 and CaMKII in the ‘learning ganglia’. Top set of panels: example from the buccal ganglia, bottom set of panels: example from the cerebral ganglia. GluA1 (green) and CaMKII (red) fluorescent signal is shown in the same section. The pT305-CaMKII signal (originally green, but pseudocoloured in blue here) is shown in the sections consecutive to the ones in which the GluA1 and CaMKII signal was detected. GluA1 and CaMKII are ubiquitously expressed in the neuronal somata of the same sections from both the buccal and cerebral ganglia. GluA1 and pT305-CaMKII are both strongly expressed in the neuropile (asterisks). Arrows indicate examples of neuronal cell bodies with particularly strong colocalization of GluA1 with CaMKII and also showing strong pT305-CaMKII expression in the consecutive section. The CaMKII content of the neuropile is smaller compared with that of the neuronal cell bodies. Scale bars represent 50 μm. This experiment was replicated three times. Figure 5: Colocalization of GluA1 and CaMKII in the ‘learning ganglia’. Top set of panels: example from the buccal ganglia, bottom set of panels: example from the cerebral ganglia. GluA1 (green) and CaMKII (red) fluorescent signal is shown in the same section. The pT305-CaMKII signal (originally green, but pseudocoloured in blue here) is shown in the sections consecutive to the ones in which the GluA1 and CaMKII signal was detected. GluA1 and CaMKII are ubiquitously expressed in the neuronal somata of the same sections from both the buccal and cerebral ganglia. GluA1 and pT305-CaMKII are both strongly expressed in the neuropile (asterisks). Arrows indicate examples of neuronal cell bodies with particularly strong colocalization of GluA1 with CaMKII and also showing strong pT305-CaMKII expression in the consecutive section. The CaMKII content of the neuropile is smaller compared with that of the neuronal cell bodies. Scale bars represent 50 μm. This experiment was replicated three times. Full size image We found that similar to GluA1 levels ( Fig. 2a ), levels of pT305-CaMKII were significantly increased at 6 h post conditioning in samples comprising the buccal and cerebral ganglia and the cerebro-buccal connectives from the paired as well as the unpaired groups of animals compared with the naive controls ( Fig. 6a ). However, unlike the samples from the paired training group, the level of pT286-CaMKII was significantly lower than baseline in the samples from the unpaired group ( Fig. 6b ) that showed no response to the CS ( Figs 1 and 2b ). Taken together, these data suggested that for associative memory at 24 h after training, both an elevated level of pT305-CaMKII and at least a baseline level of pT286-CaMKII are required during the period of ongoing memory consolidation at 6 h post training. 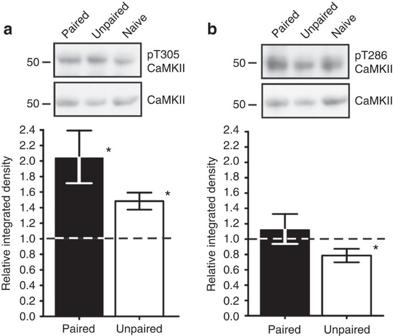Figure 6: Effects of training on T305 and T286 phosphorylation of CaMKII during memory consolidation. Samples (each containing homogenates of 12 pairs of buccal and cerebral ganglia plus the cerebro-buccal connectives) from three groups of animals, Paired, Unpaired and Naive, were used in each replicate experiment. Examples of immunoblot bands shown above the graphs. Full-length blots are shown inSupplementary Fig. 7b,c. The means (±s.e.m.) of pT305-CaMKII (a) or pT286-CaMKII (b) over CaMKII levels are shown (relative integrated density). The values thus calculated for paired samples (a,N=13;b,N=11) and unpaired samples (a,N=13;b,N=11) were normalized to the mean of the values obtained from naive samples (a,N=13; b,N=11), providing a baseline value of 1 (dashed lines). Both paired and unpaired training similarly increases the level of pT305-CaMKII 6 h after training (a, one-samplet-tests: Paired versus baseline,P<0.02; Unpaired versus baseline,P<0.004. Asterisks indicate significant differences compared with the baseline. Two-samplet-test: Paired versus Unpaired group,P=0.09). Unlike T305 phosphorylation, T286 phosphorylation remains unaffected by paired training (b, one-samplet-test: Paired versus baseline,P=0.56) and is significantly reduced by unpaired training (b, one-samplet-test: Unpaired versus baseline,P<0.04). These experiments were replicated twice. Figure 6: Effects of training on T305 and T286 phosphorylation of CaMKII during memory consolidation. Samples (each containing homogenates of 12 pairs of buccal and cerebral ganglia plus the cerebro-buccal connectives) from three groups of animals, Paired, Unpaired and Naive, were used in each replicate experiment. Examples of immunoblot bands shown above the graphs. Full-length blots are shown in Supplementary Fig. 7b,c . The means (±s.e.m.) of pT305-CaMKII ( a ) or pT286-CaMKII ( b ) over CaMKII levels are shown (relative integrated density). The values thus calculated for paired samples ( a , N =13; b , N =11) and unpaired samples ( a , N =13; b , N =11) were normalized to the mean of the values obtained from naive samples ( a , N =13; b, N =11), providing a baseline value of 1 (dashed lines). Both paired and unpaired training similarly increases the level of pT305-CaMKII 6 h after training ( a , one-sample t -tests: Paired versus baseline, P< 0.02; Unpaired versus baseline, P< 0.004. Asterisks indicate significant differences compared with the baseline. Two-sample t -test: Paired versus Unpaired group, P= 0.09). Unlike T305 phosphorylation, T286 phosphorylation remains unaffected by paired training ( b , one-sample t -test: Paired versus baseline, P= 0.56) and is significantly reduced by unpaired training ( b , one-sample t -test: Unpaired versus baseline, P< 0.04). These experiments were replicated twice. Full size image Next, the necessity for an elevated level of pT305-CaMKII in the consolidation of long-term memory was investigated in an experiment using three groups of animals: paired and CaMKIINtide-treated, paired and vehicle-treated and naive ( Fig. 7a ). It was not necessary to use an unpaired group in this experiment because our previous experiments showed that animals in this control group did not respond to the CS and therefore the link between pharmacological treatments and inhibition of the conditioned response cannot be studied in them. 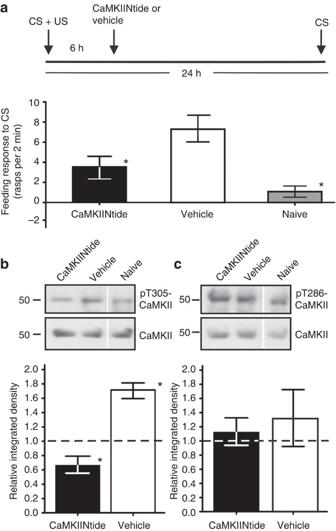Figure 7: pT305-CaMKII and memory consolidation inLymnaea. (a) Timeline for the behavioural experiment (conducted concurrently with the biochemical assays shown inbandc) is shown above the diagram. The classically conditioned and CaMKIINtide-treated animals (N=23) as well as the Naive animals (N=16) showed a significantly lower (asterisks) feeding response to the CS compared with the classically conditioned vehicle-treated animals (N=21). One-way ANOVA:P<0.0001. Tukey’s tests: CaMKIINtide and Naive versus Vehicle, bothP<0.05, CaMKIINtide versus Naive,P>0.05. (b,c) The selective effects of CaMKIINtide on T305 phosphorylation of CaMKII. Examples of western blot bands are shown above the graphs (full-length blots inSupplementary Fig. 7d,e). The means (±s.e.m.) of pT305-CaMKII (b) or pT286-CaMKII (c) over CaMKII levels are shown (relative integrated density). Total CaMKII levels were not significantly different among the groups. The values thus calculated for each CaMKIINtide-treated (b,N=7;c,N=7) and vehicle-treated sample (b,N=6;c,N=6) were normalized to the mean of the density values obtained from the naive samples (b,N=14;c,N=12), providing a baseline of 1 (dashed line). Vehicle treatment 6 h after paired training leaves the significantly raised level of pT305-CaMKII (seeFig. 6a) unaffected, whereas CaMKIINtide treatment significantly decreases it (b). Asterisks indicate significant differences both compared to the Naive baseline and between the two paired groups. One-samplet-tests: CaMKIINtide and Vehicle versus baseline, bothP<0.03. Two-samplet-test: CaMKIINtide versus Vehicle,P<0.002. T286 phosphorylation remains unaffected by treatment with either vehicle or CaMKIINtide (c). One-samplet-tests: CaMKIINtide and Vehicle versus baseline,P=0.70 and 0.69, respectively. Two-samplet-tests: CaMKIINtide versus Vehicle,P=0.90. These experiments were replicated twice. Figure 7: pT305-CaMKII and memory consolidation in Lymnaea . ( a ) Timeline for the behavioural experiment (conducted concurrently with the biochemical assays shown in b and c ) is shown above the diagram. The classically conditioned and CaMKIINtide-treated animals ( N =23) as well as the Naive animals ( N =16) showed a significantly lower (asterisks) feeding response to the CS compared with the classically conditioned vehicle-treated animals ( N =21). One-way ANOVA: P <0.0001. Tukey’s tests: CaMKIINtide and Naive versus Vehicle, both P <0.05, CaMKIINtide versus Naive, P >0.05. ( b , c ) The selective effects of CaMKIINtide on T305 phosphorylation of CaMKII. Examples of western blot bands are shown above the graphs (full-length blots in Supplementary Fig. 7d,e ). The means (±s.e.m.) of pT305-CaMKII ( b ) or pT286-CaMKII ( c ) over CaMKII levels are shown (relative integrated density). Total CaMKII levels were not significantly different among the groups. The values thus calculated for each CaMKIINtide-treated ( b , N =7; c , N =7) and vehicle-treated sample ( b , N =6; c , N =6) were normalized to the mean of the density values obtained from the naive samples ( b , N =14; c , N =12), providing a baseline of 1 (dashed line). Vehicle treatment 6 h after paired training leaves the significantly raised level of pT305-CaMKII (see Fig. 6a ) unaffected, whereas CaMKIINtide treatment significantly decreases it ( b ). Asterisks indicate significant differences both compared to the Naive baseline and between the two paired groups. One-sample t -tests: CaMKIINtide and Vehicle versus baseline, both P <0.03. Two-sample t -test: CaMKIINtide versus Vehicle, P <0.002. T286 phosphorylation remains unaffected by treatment with either vehicle or CaMKIINtide ( c ). One-sample t -tests: CaMKIINtide and Vehicle versus baseline, P =0.70 and 0.69, respectively. Two-sample t -tests: CaMKIINtide versus Vehicle, P =0.90. These experiments were replicated twice. Full size image Twenty-four hours after conditioning, associative memory was found to be significantly impaired in the group treated with CaMKIINtide at 6 h post training compared with the vehicle-treated group ( Fig. 7a ); in fact, the mean feeding response of the CaMKIINtide-treated animals was not significantly different from that of the naive animals ( Fig. 7a ). In the same time window we detected an increased training-induced autophosphorylation of CaMKII at T305 ( Fig. 7b , Vehicle group) as well as an increased level of AMPA receptor proteins in the ‘learning ganglia’ ( Fig. 2a ). In contrast to the vehicle-treated animals (showing no impairment of memory in the concurrent behavioural test, Fig. 7a ) the western blot experiment shown in Fig. 7b revealed a significantly reduced level of pT305-CaMKII in the CaMKIINtide-treated animals (showing impaired memory in the concurrent behavioural test, Fig. 7a ), compared against both the naive baseline and the level measured in the vehicle-injected group. Importantly, in the same time window the level of pT286-CaMKII was not affected either by classical conditioning at 0 h (vehicle-injected paired group, Fig. 7c ) or by CaMKIINtide treatment at 6 h post training ( Fig. 7c ). Further, there was no statistically significant difference between the normalized pT286-CaMKII data from the CaMKIINtide and vehicle group ( Fig. 7c ). These data further indicated the selective involvement of increased CaMKII autophosphorylation at T305 in AMPA-dependent consolidation of associative memory. CaMKIINtide has been shown to inhibit both Ca 2+ -stimulated and autonomous substrate phosphorylation by CaMKII as well as autophosphorylation at T305 (ref. 35 ). The data shown in Fig. 7c already demonstrated the lack of increased levels of pT286-CaMKII at 6 h after classical conditioning as well as provided evidence for a lack of effect of CaMKIINtide on pT286-CaMKII in the same time window. To exclude the possibility that CaMKIINtide-injected at 6 h post training impairs memory consolidation by inhibiting fresh intrinsic activation of CaMKII, as it does when injected 24 h after training [24] , we injected KN-62 into a different group of animals at 6 h post training. KN-62 inhibits fresh activation of CaMKII (by affecting the interaction between the Ca 2+ /CaM complex and CaMKII) but, unlike CaMKIINtide, KN-62 does not affect the already autophosphorylated enzyme [35] , [36] . In contrast to the findings obtained with CaMKIINtide injection ( Fig. 7a ), injection with KN-62 at 6 h did not cause memory impairment at 24 h post training ( Supplementary Fig. 4a ) and it did not reduce the level of pT305-CaMKII either ( Supplementary Fig. 4b ). In the same experiment, no differences were detected in pT286-CaMKII levels among the naive and vehicle or KN-62-treated trained animals ( Supplementary Fig. 4c ), further confirming the lack of involvement of pT286-related substrate phosphorylation by CaMKII in the memory consolidation process at 6 h post training. Finally, by treating classically conditioned animals with the NMDA inhibitor MK-801 (2 μm final concentration) or its vehicle (DMSO, 0.067% final concentration) at 6 h post training and testing memory at 24 h we established that NMDA receptors do not play a role in memory consolidation at this time point ( Supplementary Fig. 5 ). Thus, although CaMKIINtide is known to affect the NMDA binding ability of CaMKII (ref. 35 ), it does not affect memory consolidation in Lymnaea via this mechanism. The behavioural and biochemical effects of CaMKIINtide observed at this time point were therefore most likely due to the demonstrated significant inhibition of CaMKII autophosphorylation at T305. Reduced AMPAR levels after CaMKIINtide treatment The behavioural results presented in the previous sections demonstrated that both CNQX and CaMKIINtide injection at 6 h post training impair long-term memory in a similar manner: they both reduced the conditioned response by around half (compare Figs 1 and 7a ). In the same time window we detected an increased training-induced autophosphorylation of CaMKII at T305 ( Figs 6a and 7b ) as well as an increased level of AMPAR proteins in the ‘learning ganglia’ ( Figs 2a and 4 ). Furthermore, we found that CaMKIINtide treatment at 6 h post training reduced the level of pT305-CaMKII ( Fig. 7b ) without affecting the level of pT286-CaMKII ( Fig. 7c ), which was also unaffected by paired training 6 h previously ( Fig. 6b ). These findings together indicated a possible link between increased pT305-CaMKII and AMPA receptor levels. In the next experiment therefore we directly tested the effect of inhibiting CaMKII T305 autophosphorylation by CaMKIINtide on learning-induced AMPAR levels. We used the western blot method in these experiments because it allows a greater statistical power compared with immunohistochemistry when testing the combined effects of training and drug treatment. When CaMKIINtide was administered at 6 h post conditioning and immunoblotting tests were performed 30 min later, we found a significant decrease, back to naive baseline level, in GluA1 expression compared with the vehicle-injected paired group in the same experiment ( Fig. 8 ). There was also a statistically significant difference between the normalized data from the CaMKIINtide and vehicle group. This result indicated a link between pT305-CaMKII and the maintenance of increased AMPAR levels. The apparent rapid removal (within 30 min after injection with CaMKIINtide) of previously synthesized AMPARs strongly suggested a role for pT305-CaMKII in the prevention of AMPAR protein degradation. 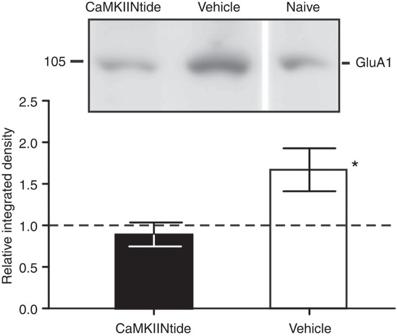Figure 8: T305 autophosphorylation of CaMKII regulates AMPAR protein levels in the ‘learning ganglia’. Example GluA1 western blot bands from a paired and CaMKIINtide-treated, a paired and vehicle-treated and a naive sample, run on the same gel, are shown above the graphs (full-length blot inSupplementary Fig. 7f). Density data obtained from CaMKIINtide (N=8) and vehicle (N=8) samples were normalized to the mean of the density data obtained from naive samples (N=8), which provided a baseline value of 1. The asterisk indicates significant difference compared with both the naive baseline and the level measured after CaMKIINtide treatment. One-samplet-tests: CaMKIINtide versus naive baseline,P=0.41 (n.s.); Vehicle versus baseline,P<0.05. Two-sample unpairedt-test: CaMKIINtide versus Vehicle,P<0.03. This experiment was replicated twice. All data presented as means±s.e.m. Figure 8: T305 autophosphorylation of CaMKII regulates AMPAR protein levels in the ‘learning ganglia’. Example GluA1 western blot bands from a paired and CaMKIINtide-treated, a paired and vehicle-treated and a naive sample, run on the same gel, are shown above the graphs (full-length blot in Supplementary Fig. 7f ). Density data obtained from CaMKIINtide ( N =8) and vehicle ( N =8) samples were normalized to the mean of the density data obtained from naive samples ( N =8), which provided a baseline value of 1. The asterisk indicates significant difference compared with both the naive baseline and the level measured after CaMKIINtide treatment. One-sample t -tests: CaMKIINtide versus naive baseline, P =0.41 (n.s. ); Vehicle versus baseline, P <0.05. Two-sample unpaired t -test: CaMKIINtide versus Vehicle, P <0.03. This experiment was replicated twice. All data presented as means±s.e.m. Full size image Proteasomal inhibition rescues both AMPAR levels and ALTM The hypothesis that CaMKIINtide-induced downregulation of pT305-CaMKII impairs LTM and reduces AMPAR levels via proteasomal activity was tested in an experiment where we investigated whether the use of the reversible proteasomal inhibitor MG132 could offset the behavioural and biochemical effects of CaMKIINtide on LTM and AMPAR levels, respectively. We reasoned that if proteasomal inhibition rescued AMPAR levels from CaMKIINtide-induced reduction this would lend further support to the notion that autophosphorylation of CaMKII at T305 was an important factor in maintaining them in the face of proteasomal degradation. In this experiment we used five groups of classically conditioned and one group of naive animals. Six hours after classical conditioning, the first group of trained animals was left untreated, the second group was injected with vehicle, the third group was injected with MG132, the fourth group was injected with CaMKIINtide, while the fifth trained group was injected with a mixture of CaMKIINtide and MG132. When the trained animals were tested with the CS 24 h after conditioning (and 18 h after injection when drugs or vehicle was administered) and also compared against a naive control group, an ANOVA indicated a source of significant difference among the six groups ( Fig. 9a ). Post hoc tests showed that the CaMKIINtide-injected group gave a significantly weaker feeding response to the CS than any of the other trained groups with the response only being marginally higher than the CS response in the naive control group. The most important finding of this experiment however was that when CaMKIINtide was injected together with MG132, memory impairment did not occur at 24 h after training, confirming that proteasomal inhibition can rescue memory from the impairment caused by inhibition of CaMKII autophosphorylation at T305. Interestingly, treatment with MG132 alone seemed to have a mild boosting effect on memory 18 h later, although this was not significant. 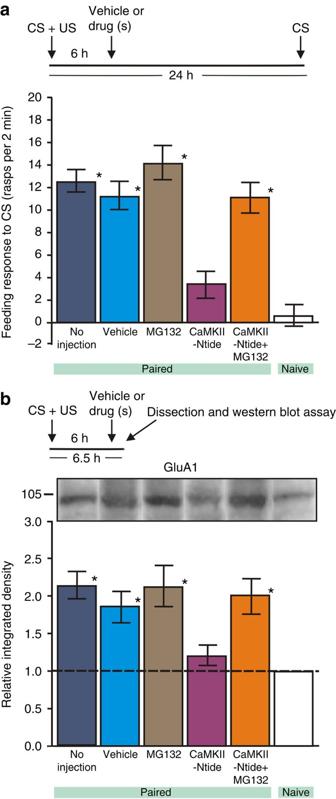Figure 9: Proteosome inhibition offsets CaMKIINtide-induced memory impairment and the decrease in AMPARs. (a) MG132 co-injected with CaMKIINtide at 6 h post training rescues ALTM. Untreated paired (no injection,N=24), DMSO-injected (Vehicle,N=12), MG132-injected (N=12) and CaMKIINtide+MG132-injected (N=12) all showed significantly higher feeding responses to the CS compared with CaMKIINtide-injected (N=24) and naive (N=24) animals. Asterisks indicate significantly higher feeding responses to the CS compared with CaMKIINtide and naive levels. ANOVA:P<0.001. Tukey’s test: CaMKIINtide-injected versus all other trained groups,P<0.05; CaMKIINtide-injected versus Naive group,P>0.05; CaMKIINtide+MG132-injected group versus CaMKIINtide-injected and Naive group, bothP<0.05. (b) MG132 co-injected with CaMKIINtide at 6 h post training rescues GluA1 receptor levels. Samples from untreated paired (no injection,N=4), DMSO-injected (Vehicle,N=8), MG132-injected (N=8) and CaMKIINtide+MG132 injected (N=8) animals all showed significantly higher GluA1 levels compared with CaMKIINtide-injected (N=8) and naive (N=8) animals. Full-length blot is shown inSupplementary Fig. 8. Asterisks indicate significantly higher relative integrated density values compared with CaMKIINtide and naive baseline level, respectively. One-way ANOVA:P<0.006. Tukey's: CaMKIINtide-injected versus all other trained groups,P<0.05. One-samplet-tests: CaMKIINtide-injected versus naive baseline,P>0.05; all other groups versus naive baseline,P<0.05. These experiments were replicated twice. All data presented as means±s.e.m. Figure 9: Proteosome inhibition offsets CaMKIINtide-induced memory impairment and the decrease in AMPARs. ( a ) MG132 co-injected with CaMKIINtide at 6 h post training rescues ALTM. Untreated paired (no injection, N =24), DMSO-injected (Vehicle, N =12), MG132-injected ( N =12) and CaMKIINtide+MG132-injected ( N =12) all showed significantly higher feeding responses to the CS compared with CaMKIINtide-injected ( N =24) and naive ( N =24) animals. Asterisks indicate significantly higher feeding responses to the CS compared with CaMKIINtide and naive levels. ANOVA: P <0.001. Tukey’s test: CaMKIINtide-injected versus all other trained groups, P <0.05; CaMKIINtide-injected versus Naive group, P >0.05; CaMKIINtide+MG132-injected group versus CaMKIINtide-injected and Naive group, both P <0.05. ( b ) MG132 co-injected with CaMKIINtide at 6 h post training rescues GluA1 receptor levels. Samples from untreated paired (no injection, N =4), DMSO-injected (Vehicle, N =8), MG132-injected ( N =8) and CaMKIINtide+MG132 injected ( N =8) animals all showed significantly higher GluA1 levels compared with CaMKIINtide-injected ( N =8) and naive ( N =8) animals. Full-length blot is shown in Supplementary Fig. 8 . Asterisks indicate significantly higher relative integrated density values compared with CaMKIINtide and naive baseline level, respectively. One-way ANOVA: P <0.006. Tukey's: CaMKIINtide-injected versus all other trained groups, P <0.05. One-sample t -tests: CaMKIINtide-injected versus naive baseline, P >0.05; all other groups versus naive baseline, P <0.05. These experiments were replicated twice. All data presented as means±s.e.m. Full size image To investigate the link between the behavioural findings and changes in AMPAR levels we used the same types of trained and naive groups as before in an experiment in which we used western blotting to measure changes in GluA1 expression after treatment with CaMKIINtide and MG132 at 6 h post training. The findings of this experiment mirrored those of the behavioural tests. AMPAR levels were significantly reduced by treatment with CaMKIINtide alone but were normal when CaMKIINtide was co-applied with MG132 ( Fig. 9b ). To investigate the time windows in which the administration of MG132 can rescue the 24 h memory from CaMKIINtide-induced impairment, we performed two further experiments. In one experiment administration of MG132 preceded that of CaMKIINtide by 1 h and in another experiment it followed the administration of CaMKIINtide by 1 h. These experiments showed that injection with MG132 at 5 h had a similar memory-rescuing effect on trained animals treated with CaMKIINtide at 6 h post training ( Fig. 10a ) as when the two drugs were co-injected at 6 h post training. However, when MG132 was administered with a 1-h delay after CaMKIINtide treatment at 6 h it was no longer effective in rescuing long-term memory ( Fig. 10b ). 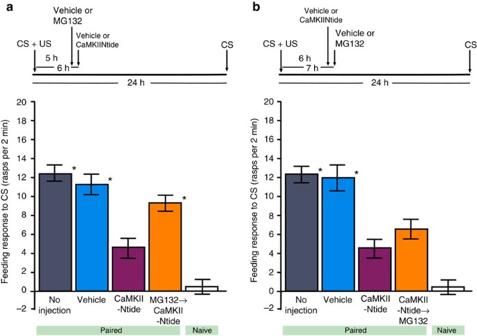Figure 10: Proteasome inhibition 1 h before but not 1 h after CaMKIINtide treatment offsets memory impairment. (a) MG132 injected 1 h before treatment with CaMKIINtide at 6 h post training offsets the effect of CaMKIINtide on LTM. Untreated paired (no injection,N=22), DMSO-injected (Vehicle,N=14), and MG132→CaMKIINtide-injected (N=15) groups of animals all showed significantly higher feeding responses to the CS compared with CaMKIINtide-injected (N=23) and naive (N=22) animals. (b) MG132 injected 1 h after CaMKIINtide treatment at 6 h post training does not offset the effect of CaMKIINtide on LTM. The untreated paired (no injection,N=22) and DMSO-injected (Vehicle,N=13) groups of animals showed significantly higher feeding responses to the CS compared with CaMKIINtide-injected (N=23), CaMKIINtide→MG132 injected and naive (N=23) animals. Asterisks indicate significantly higher feeding responses to the CS compared with CaMKIINtide and naive levels in (a) and CaMKIINtide, CaMKIINtide→MG132 and naive levels in (b) (ANOVAs,P<0.001; Tukey’s,P<0.05). These experiments were replicated twice. All data are presented as means±s.e.m. Figure 10: Proteasome inhibition 1 h before but not 1 h after CaMKIINtide treatment offsets memory impairment. ( a ) MG132 injected 1 h before treatment with CaMKIINtide at 6 h post training offsets the effect of CaMKIINtide on LTM. Untreated paired (no injection, N =22), DMSO-injected (Vehicle, N =14), and MG132→CaMKIINtide-injected ( N =15) groups of animals all showed significantly higher feeding responses to the CS compared with CaMKIINtide-injected ( N =23) and naive ( N =22) animals. ( b ) MG132 injected 1 h after CaMKIINtide treatment at 6 h post training does not offset the effect of CaMKIINtide on LTM. The untreated paired (no injection, N =22) and DMSO-injected (Vehicle, N =13) groups of animals showed significantly higher feeding responses to the CS compared with CaMKIINtide-injected ( N =23), CaMKIINtide→MG132 injected and naive ( N =23) animals. Asterisks indicate significantly higher feeding responses to the CS compared with CaMKIINtide and naive levels in ( a ) and CaMKIINtide, CaMKIINtide→MG132 and naive levels in ( b ) (ANOVAs, P <0.001; Tukey’s, P <0.05). These experiments were replicated twice. All data are presented as means±s.e.m. Full size image In this study, we tested the hypothesis that pT305-CaMKII plays a role in the maintenance of increased AMPA type glutamate receptor levels after classical conditioning. Using a combination of single-trial food-reward classical conditioning, pharmacological treatments, western blot assays and immunohistochemistry in Lymnaea , we show that (i) both GluA1 receptor protein and pT305-CaMKII levels are increased at 6 h post training; (ii) inhibition of GluA1 receptor activation or inhibition of CaMKII T305 autophosphorylation at the same time point impairs ongoing memory consolidation. Importantly, we also show that at 6 h after classical conditioning there is neither residual (autonomous) nor new (Ca 2+ /CaM-triggered) T286 phosphorylation above naive control levels, which would enable a higher-than-baseline level of CaMKII activation and resulting increased phosphorylation of substrates that are important for plasticity (for example, AMPA receptors [37] and CPEB [38] ). Therefore, neither the reduced GluA1 level nor the memory impairment by CaMKIINtide applied at this time point to classically conditioned animals was due to reduced pT286-CaMKII levels. The observation that NMDA receptor activity is not required for ongoing memory consolidation at 6 h post training also rules out that the observed effects were due to the NMDA-binding site of CaMKII being blocked by CaMKIINtide. Thus, the most likely explanation for the CaMKIINtide-induced decrease in GluA1 expression and memory impairment is that it was the result of the demonstrated reduced autophosphorylation of CaMKII at T305. We also compared the GluA1 receptor protein content of the ‘learning ganglia’ in snails treated with CaMKIINtide or vehicle or a mixture of CaMKIINtide and the proteasomal inhibitor MG132 at 6 h after classical conditioning. Not only did these experiments establish a strong correlative link between pT305-CaMKII and maintained AMPAR levels but they also showed that the inhibition of proteasomal activity offsets the deleterious effects of CaMKIINtide on both GluA1 levels and memory. These experiments therefore provided the first evidence for a link between pT305-CaMKII and maintained increased levels of GluA1 receptor protein, which were shown to occur in parallel during the period of memory consolidation and also were shown to be necessary for the consolidation of long-term memory in the same period. Previous studies already have shown that one of the ways that CaMKII plays its complex multiple roles in synaptic plasticity and learning and memory is via the regulation of AMPAR expression and function [9] , [39] , [40] . The present study significantly extends these previous findings by suggesting a major new role for pT305-CaMKII in AMPA-dependent memory consolidation. Previous work also has shown that not only is the initial T286 autophosphorylation of CaMKII important for the phosphorylation of AMPARs [8] , [41] , [42] , it is also essential for the recruitment of the proteasome [14] , which in turn plays a role in the degradation of the components of the AMPAR complex following training [43] . Previous work has suggested a number of important functions for the autophosphorylation of CaMKII at T305 in the acquisition phase of various different learning tasks and synaptic plasticity, and even in metaplasticity and certain neurological disorders, such as Angelman syndrome [44] , [45] . However, our study is the first demonstration of the importance of this inhibitory autophosphorylation and its maintenance for memory consolidation after classical conditioning. What makes this new finding particularly significant is that this novel role for pT305-CaMKII is also linked to the regulation of AMPAR function. Our combined proteasomal and pT305-CaMKII inhibition experiments suggest that there is a dynamic and temporally controlled interaction between inhibitory CaMKII autophosphorylation, proteasomal activity and AMPARs during memory consolidation. The detailed biochemical mechanisms by which pT305-CaMKII contributes to the maintenance of AMPAR levels remains to be determined; however, we hereby propose a hypothesis based on our findings from the proteasomal inhibition experiments, together with information from previous work. Importantly, autonomously active pT286-CaMKII plays a dual role in both the recruitment of the proteasome to the PSD and its activation immediately following training [14] . Both of these processes promote the degradation of synaptic proteins, including agonist-activated ubiquitinated AMPARs [8] . Despite this apparent early proteasomal degradation of AMPARs, their levels were found to be high at 6 h post training both in our experiments and previous experiments in mice [17] . Nevertheless, another previous key observation helped us to identify a likely link between CaMKII and maintained AMPAR levels: inhibitory autophosphorylation of CaMKII at T305 promotes its dissociation from the PSD [19] , [20] and therefore presumably from the proximity of the proteasome originally recruited to the PSD by pT286-CaMKII (ref. 14 ). Based on this information and the observations described in the present study, we propose that during the AMPAR activation-dependent consolidation phase of memory formation, T305 phosphorylation of CaMKII reverses the initial effects of pT286-CaMKII on the proteasome and thus leads to the reduction of proteasomal degradation of AMPARs in synapses. This novel mechanism may provide a means for bidirectional regulation of learning-increased AMPAR levels by CaMKII, with T286 autophosphorylation promoting their downregulation shortly after learning and T305 autophosphorylation promoting their maintenance during memory consolidation. The proposed link between pT305-CaMKII and AMPAR levels does not rule out that there are mechanisms of AMPA-dependent memory consolidation in Lymnaea that are independent from pT305-CaMKII. This possibility was strongly indicated by the finding that even though CaMKIINtide treatment at 6 h post training decreases pT305-CaMKII levels to below baseline ( Fig. 7c ), it does not lead to full memory erasure at 24 h post training ( Fig. 7a ). Another strong candidate molecule for maintaining elevated synaptic levels of AMPARs following learning in both vertebrates and invertebrates is PKM, the catalytically active fragment of atypical PKC [46] , [47] . A role for PKM has recently been reported for early consolidation of intermediate (translation-dependent, <4 h post training) but not long-term (transcription-dependent, >4 h post training) memory in Lymnaea [48] , using the same single-trial paradigm that we used in the current study. We cannot however rule out that PKM is involved in intermediate or late term consolidation/maintenance of LTM in Lymnaea and therefore at 6 h post training PKM and pT305-CaMKII may be playing complementary roles in maintaining elevated GluA1 levels for ongoing memory consolidation. Currently, we can only speculate on the exact role of GluA1 activity in the ongoing processes of memory consolidation in Lymnaea . Recent work in humans has shown that an offline activation of glutamatergic synapses seems to play a critical part in the consolidation of memory in the visual cortex [49] . In rats, AMPARs in the perirhinal cortex mediate consolidation as well as encoding and retrieval of object recognition memory [50] . There is also evidence of the involvement of AMPARs in consolidation of associative memory in the chick, taking place several hours after a one-trial passive avoidance task [51] . This latter finding is most directly comparable to our findings, which are also based on a single-trial classical conditioning paradigm. These results therefore suggest that the role of AMPARs in ongoing memory consolidation is an evolutionarily conserved one, which, as shown here for the first time, is dependent on the T305 autophosphorylation of another highly conserved key signalling molecule of memory function, CaMKII, via its interaction with the proteasome. Experimental animals Lymnaea stagnalis pond snails, bred at the University of Sussex, were maintained in large holding tanks using Cu 2+ -free water (also used throughout all the experiments) at 18–20 °C with a 12-h light–dark cycle, with ad libitum lettuce and fish food (TETRA Werke, Melle, Germany). The animals used in the experiments were between 3 and 4 months old and they were food-deprived for 2 days before the beginning of the conditioning procedure. Single-trial conditioning and pharmacological treatments We used an established single-trial food-reward classical conditioning protocol that leads to the formation of transcription- and translation-dependent long-term associative memory in Lymnaea [22] , [23] , [25] , [34] , [52] . This paradigm also has been used previously to elucidate the role of pT286-CaMKII in learning and late memory consolidation in Lymnaea [24] . Briefly, following a 10-min acclimatization period in a Petri dish containing 90 ml of water, snails were presented with conditioned and unconditioned stimuli (CS and US) in a paired or unpaired manner. In the paired training protocol, 5 ml of amyl acetate solution (0.08% in water, the CS) was delivered into the dish, followed after a 30-s interval by 5 ml of sucrose solution (13.4% in water, the US). In the unpaired protocol, the CS was followed by the US with a 1-h interval. Following training, snails were transferred back to their home tanks after a 10-min period in a tank of clean water. For behavioural pharmacological experiments, animals were injected with CaMKIINtide (final concentration 4 μM in 0.17% DMSO in the haemolymph; Merck Chemicals Ltd, Nottingham, UK), a specific inhibitor of CaMKII and an inhibitor of autophosphorylation of CaMKII at T305 (ref. 35 ), with CNQX (final concentration 20 μM in the haemolymph), a selective antagonist of AMPARs, or with MG132, a reversible proteasome inhibitor (final concentration 1 μM in the haemolymph) at 6 h post conditioning. The use of MG132 was based on a recent study in which it was successfully used in associative learning experiments with intact honeybees to test the role of protein degradation in memory consolidation [53] . Neither of these drugs affected the animals’ ability to generate a full feeding motor programme in response to food 18 h after injection ( Supplementary Fig. 6 ). For concurrently conducted behavioural and immunoblotting experiments, animals were treated with CaMKIINtide, MG132 or both, or with the DMSO-containing vehicle, at 6 h after paired or unpaired training and dissected 30 min later. The cerebral and buccal ganglia were collected and frozen immediately on dry ice for further processing and immunoblotting. During behavioural testing, which took place 24 h after acquisition in all experiments, individual snails from the different experimental and control groups were placed into Petri dishes using a blind procedure. After a 10-min acclimatization period, spontaneous rasps (stereotyped feeding movements of the mouth) were counted for 2 min. Following the delivery of CS, rasps were counted for a further 2 min. The feeding response to the CS was defined as the difference between the number of rasps in the presence of CS and the number of spontaneously occurring rasps. Identification of a mammalian GluA1-like protein in Lymnaea The cloning and sequence analysis of a GluA-like gene from the pond snail Lymnaea stagnalis by Hutton et al. [54] predicted a mature peptide with 898 amino acids and an N-terminal signal peptide [55] with 19 amino acids. The predicted size of this GluA1-like protein was about ~101 kDa; further hydrophobic analysis of this sequence clearly revealed the presence of three strongly hydrophobic regions that correspond to the TM1, TM3 and TM4 transmembrane regions of vertebrate ionotropic glutamate receptor subunits [54] , [56] . This mature peptide, which was subsequently named Lym-eGluR1 (ref. 57 ), shares substantial amino-acid sequence homology with mammalian AMPA-selective subunits, and more than with other selective subunits. Based on this evidence of sequence homology between Lym-eGluR1 and the mammalian GluA1-AMPA subunit, we chose a mammalian antibody selective for GluA1-AMPA, ab31232 (from rabbit), along with its corresponding synthetic peptide, ab28424 (Abcam, UK), to detect Lym-eGluR1 expression and optimize the use of this mammalian antibody for Lymnaea protein samples. To test the mammalian primary antibody, protein samples were prepared from mouse hippocampus and from Lymnaea whole brains, resolved by sodium dodecyl sulphate (SDS)–PAGE (8.25%) and electro-blotted on PVDF membrane. Electro-blotted membranes with resolved proteins were then subjected to immunoassays as follows. The blotted PVDF membrane was cut into three strips (across the colour marker, CM lanes). Each strip always contained imprints of at least one set of mouse and Lymnaea resolved proteins and they were exposed to different immunoassay applications. All membrane strips were blocked for 1 h at room temperature (RT) in Tris-buffered saline (TBS) containing 0.15% Tween 20 with 3% non-fat dry milk. One strip of membrane was incubated overnight at 4 °C with the ab31232 antibody (1/1,000 w / v at 0.5 μg μl −1 ) in blocking solution (TBS/Tween 20/milk). A second strip of membrane containing the same set of mouse and Lymnaea imprints was incubated overnight at 4 °C in a ‘cocktail’ designed to block the primary antibody: ab31232 was used at the same concentration (1/1,000 w / v at 0.5 μg μl −1 ) together with a 15-fold higher concentration of the synthetic peptide ab28424 (1/66.6 w / v at 1 μg μl −1 ). The third control strip of samples was not exposed to any primary antibody or synthetic peptide. All membrane strips were washed in TBS/Tween 20 three times, and incubated for 1.5 h at RT with secondary antibody (1:1,000 HRP-linked anti-rabbit IgG antibody, Cell Signalling, UK) diluted in TBS/Tween 20/milk. All membranes were then washed and protein bands were visualized using enhanced chemiluminescence substrates (Millipore) ( Supplementary Fig. 1a ). Control strips were only probed with the secondary antibody and showed no bands ( Supplementary Fig. 1b , ‘Controls’). All western blot and immunoassays mentioned above with the selective antibody and its corresponding synthetic peptide were performed four times with mouse and Lymnaea samples. The western blot and immunoassay with rabbit ab3123 clearly identified the mouse GluA1 band slightly lower than 100 kDa (~98 kDa) as also described by the manufacturers. Importantly, it showed corresponding bands in Lymnaea samples, one at 98 kDa and another, much more intense band at ~105 kDa ( Supplementary Fig. 1a ). When the same primary antibody was pre-incubated with the synthetic peptide in the second strip, the expression of mouse GluA1 at 98 kDa was suppressed significantly and so were the corresponding bands in the Lymnaea samples ( Supplementary Fig. 1b ). In the Lymnaea samples, a number of other bands were also detected by the antibody, although no significant corresponding mouse bands were found; these may be due to non-specific cross reactivity of some Lymnaea proteins with the mammalian primary antibody. These bands also became weaker after pre-incubation but the largest reduction in intensity was detected on the ~98 kDa and ~105 kDa bands. From the above observations it can be concluded that the mammalian GluA1 primary antibody is most specific to Lymnaea bands of ~100 kDa, most prominently at 105 kDa. Western blot assays after classical conditioning Protein homogenates for immunoblotting were prepared from the pooled cerebral and buccal ganglia and cerebro-bucal connectives of 12 snails per sample (conducted in parallel with behavioural testing on different groups of animals trained at the same time). We assayed CaMKII and pT286-CaMKII as well as pT305-CaMKII levels with mammalian antibodies in Lymnaea nervous tissue based on a methodology we developed in a previous study [24] . The buccal and cerebral ganglia (interconnected by the cerebro-buccal connective) were dissected and prepared as protein samples for western blotting. After homogenization in ice-cold Tris lysis buffer (125 mM TRIS, pH 6.8), the samples were put on ice, and then centrifuged at 4 °C. Supernatants were removed into a clean tube and were then boiled at 95 °C for 5 min with 50 mM Tris (pH 6.8), 2% ( w / v ) SDS, 10% glycerol, 10% β-mercaptoethanol, 0.01% bromophenol blue, 2 mM Na 3 VO 4 , 10 mM NaF, 10 mM MgCl 2 , 50 μM ATP, 8 mM EGTA and 2% protease inhibitor cocktail (Sigma-Aldrich Company Ltd, Dorset UK) and then centrifuged at 13,000 g at 4 °C to remove debris. Approximately 20 μg of each sample was run on SDS-PAGE and blotted according to standard methods. The blotted PVDF membrane was blocked for 1 h at RT or overnight at 4 °C in Tris Buffer Saline (TBS) with 0.15% Tween 20 with 5% non-fat dry milk. The membrane was incubated for 2 h at 20 °C or overnight at 4 °C with either mouse monoclonal IgG anti-α subunit CaM-kinase II (Clone 6G9, 1:2,000 v / v ), or mouse monoclonal IgG anti-phospho-CaM-kinase II (T286 (1:1,000 v / v ) and T305 (1:500 v / v ), respectively) (all from Millipore Ltd, Hertfordshire, UK), diluted in TBS/Tween 20/milk and BSA. The membrane was then washed in TBS/Tween three times, and incubated for 1 h at 20 °C with secondary antibody (1:1,000 horseradish peroxidase (HRP)-linked goat anti-rabbit or anti-mouse IgG antibody, Cell Signalling, UK) diluted in TBS/Tween 20/milk and BSA. The membrane was then washed in TBS/Tween twice and once in TBS. Protein bands were visualized using enhanced chemiluminescence (Millipore Ltd, Hertfordshire, UK). Control samples were only probed with the secondary antibody and showed no bands. Densitometric analysis was performed in a blind manner using ImageJ software. Justification of the use of a mammalian antibody to detect GluA1-like proteins in Lymnaea in the classical conditioning experiments of the present study was verified by running samples prepared from mouse hippocampus and Lymnaea nervous tissue in parallel on the same electrophoretic gels and challenging them with the same mammalian GluA1 antibody in immunoblotting tests (refer to the section ‘Identification of a mammalian GluA1-like protein in Lymnaea ’ for details). Immunohistochemistry The paired buccal and cerebral ganglia were dissected out from Paired, Unpaired and Naive groups of snails according to their corresponding group timeline, as described under the ‘Single-trial conditioning protocol and pharmacological treatments’ section. Each pair of dissected buccal and cerebral ganglia from their respective groups were immediately fixed in 4% paraformaldehyde solution for an hour at RT, followed by 30% sucrose incubation overnight at 4 °C. The following morning, all samples were soaked in OCT (embedding medium, Fisher Scientific, UK) for 5 min and then quickly frozen in liquid nitrogen (−180 °C) to prepare the sample blocks for cryosectioning. About 12 or 15-μm thick serial sections were prepared from each ganglion and dried well on slides. Later, all sample sections were washed with PBS buffer, permealized and blocked in 0.25% Triton X-100 in PBS and with 1% BSA, respectively (blocking buffer solution) for 1 h and 30 min, at RT. Primary antibodies were diluted in the above blocking buffer (before application) as follows: rabbit Anti-GluA1, 1:100 v / v (Abcam, UK); mouse anti-PSD95 antibody (clone 6G6-1C9), 1:100 v / v (Novus, UK); rabbit anti-phospho-CaMKII (Thr305), 1:100 v / v and mouse anti-CaMKII, 1:50 v / v (Millipore, UK). All primary antibody incubations were performed overnight at 4 °C, and then the sections were washed and transferred into secondary PBS-blocking solution containing 4% normal goat serum and 0.25% Triton X-100, for an hour at RT. Secondary antibodies were used at a dilution of 1:200 v / v for goat anti-rabbit IgG (Invitrogen, UK) and 1:100 v / v for goat anti-mouse IgG (Invitrogen, UK), in the above secondary blocking buffer and incubations were performed at RT for 1 h and 30 min. The goat anti-rabbit IgG and goat anti-mouse IgG, secondary antibodies were conjugated with Alexa-fluor 488 nm (green fluorescent dye) and Alexa-fluor 568 nm (red fluorescent dye) fluorophores, respectively. After secondary incubations, all sections were washed in PBS. Finally, sections on slides were mounted using the fluorescence protector Fluoroshield, with DAPI, where required (Sigma, UK). Control tests performed on alternating sections by omitting the primary antibody showed no signals or very low background noise only. Confocal microscopy The sections from the cerebral and buccal ganglia were imaged on a Carl Zeiss Laser Scanning Microscope (LSM) 510, using a × 10, 0.30 Plan-Neofluar numerical aperture objective (in single staining, whole-ganglia quantification study) or using a × 20, 0.50 Plan-Neofluar numerical aperture objective (in multiple staining, specific synaptic colocalization study). All confocal images that were used in quantification were captured by keeping all parameters, features and specification similar between the groups, to avoid any bias between the sections from different conditioning groups. For analysis, images were prepared merging three optical slices together (each from top, middle and bottom of the section). Finally, the Y projection (at 0° angle) of their respective Z stacks (~12 μm) was considered for quantification, as described below. Image analysis For the qualitative analysis of the co-localization of GluA1 and PSD-95, two techniques, Dye overlay and Threshold overlap (MacBiophotonics ImageJ, NIH), were used. The standard test for the colocalization of GluA1 and PSD-95 proteins was performed by tagging both target proteins with their respective primary and secondary antibodies conjugated with contrasting fluorescent dyes (GluA1: Alexa-fluor 488, green, PSD-95: Alexa-fluor 568, red). The green and red signals were imaged separately in their corresponding emission band of wavelengths. All images were scanned and processed through Carl Zeiss LSM Image browser application. Using the same application, the red and green channels, together with the blue channel (that represents the DAPI staining), were merged to generate multiple stained confocal images to test the colocalization of the above molecules. To visualize colocalized signals, a qualitative threshold-overlap method was used, where pixels that had both red and green values greater than 50 were highlighted with white dots in an 8-bit grey-scale (0–256) image, which was generated using MacBiophotonics ImageJ software and plug-ins (ImageJ 1.47a, NIH). For the quantitative analysis of the colocalization of GluA1 and PSD-95, the intensities of staining for the two target proteins were calculated by intensity correlation analysis (ICA), which is based on the principle explained by Li et al. [58] Briefly, if two molecules (for example, GluA1 and PSD-95) are colocalized and work as parts of the same complex, then their staining intensities in each pixel should vary in synchrony. In this case, in the majority of pixels both of their expressions should go up and down together from their respective means, and produce positive PDM values (product of their differences from the mean). However, if they do not colocalize or work as parts of different complexes, they will mostly have negative PDM values. Quantification of GluA1 levels in Lymnaea ganglia Two different approaches were used to quantify the differences in the level of GluA1 expression in the Paired, Unpaired and Naive groups. All images were obtained as described under the ‘Confocal microscopy’ subheading. Four Z stack images ( Y Projection; 0°) from the middle regions of the paired buccal ganglia, and the left and right cerebral hemiganglia were processed as 8-bit images. Pixels were analysed using MacBiophotonics ImageJ software and plug-ins (ImageJ 1.47a, NIH). In the first approach, all images were quantified following an ImageJ protocol. In this process, the percentage of the area (% area) of GluA1 expression, above a certain threshold level, was calculated over the entire area (A) of that region of the corresponding ganglia. In an image ( Z stack), the entire area of interest (region of ganglia) was selected using an image threshold that was processed based on the algorithm proposed by Otsu [59] . In this way, an outline of the area of interest was generated and almost all absolute background noise was reduced and thus omitted from all calculations. The total area under that selection was measured using the ‘Analyse Particles’ option in ImageJ (Ver-1.47a). Further, in the same 8-bit image, the threshold was raised to 65 (on a 0–255 scale), in order to avoid all low-intensity background pixels and select specific areas of GluA1 expression (with high-intensity pixels). The above procedure was applied to images of all four stacks obtained from each sample. Finally, the mean percentage area of above the threshold GluA1 expression in the buccal and cerebral ganglia was calculated for each replicate snail. This procedure was followed with the threshold maintained constant in all paired, unpaired and naive samples ( N =5 replicates in each group). In the second approach, based on calculating integrated density values (area × mean grey value), we analysed the differential expression of GluA1 in the paired and unpaired snail ganglia relative to naive levels. To achieve this, the same confocal Z-stack images that were used to calculate the percentage of stained area were processed in a similar way. However, in this case the ‘area’ and the ‘mean grey value’ only above the threshold of 65 (on the 0–256 grayscale) were considered. Finally, the individual stack ‘Integrated Density’ (IntDen) and their means were calculated for each sample. In the next step, all paired and unpaired integrated density results were normalized to the integrated densities of naive samples. Statistical analysis Sample size (number of biological replicates) was chosen based on previous studies [22] , [23] , [24] , [25] , [26] , [27] , [28] , [30] , [34] , [48] that used the same classical conditioning, pharmacological treatment, western blot and immunohistochemical protocols in Lymnaea employed in the present experiments. The GraphPad Prism (version 5) software was used for all statistical analysis. All data sets passed the Kolmogorov–Smirnoff normality test and therefore parametric tests were used for all statistical comparisons. In the biochemical experiments, one-sample t -tests were used to compare the normalized sample means of experimental groups against 1, with the mean of a naive group used as the baseline value for normalization. When comparing the means from two independent experimental groups (for example, Paired versus Unpaired), comparisons were made by two-sample t -tests. In the behavioural experiments, multiple comparisons between non-normalized means were made by one-way ANOVA followed by Tukey’s post hoc tests to determine pair-wise differences among the groups used in each experiment. Differences were considered significant at P< 0.05. An α level of 0.05 was used in all statistical tests. How to cite this article: Naskar, S. et al. pT305-CaMKII stabilizes a learning-induced increase in AMPA receptors for ongoing memory consolidation after classical conditioning. Nat. Commun. 5:3967 doi: 10.1038/ncomms4967 (2014).